FOXO3 signalling links ATM to the p53 apoptotic pathway following DNA damage DNA damage as a result of environmental stress is recognized by sensor proteins that trigger repair mechanisms, or, if repair is unsuccessful, initiate apoptosis. Defects in DNA damage-induced apoptosis promote genomic instability and tumourigenesis. The protein ataxia-telangiectasia mutated (ATM) is activated by DNA double-strand breaks and regulates apoptosis via p53. Here we show that FOXO3 interacts with the ATM–Chk2–p53 complex, augments phosphorylation of the complex and induces the formation of nuclear foci in cells on DNA damage. FOXO3 is essential for DNA damage-induced apoptosis and conversely FOXO3 requires ATM, Chk2 and phosphorylated p53 isoforms to trigger apoptosis as a result of DNA damage. Under these conditions FOXO3 may also have a role in regulating chromatin retention of phosphorylated p53. These results suggest an essential link between FOXO3 and the ATM–Chk2–p53-mediated apoptotic programme following DNA damage. All living organisms are inexorably exposed to environmental stress that cause DNA double-strand breaks (DSBs), which pose the greatest challenge to the maintenance of genomic stability in cells. Many anticancer agents also induce DSBs in cancer cells that promote cellular apoptosis. DSBs are generally recognized by sensors and transducers, containing signalling kinases, which can signal repair mechanisms or, if this fails, they trigger apoptosis. One of the most important proteins is ataxia-telangiectasia mutated (ATM), a crucial tumour suppressor, which is activated by DSBs though autophosphorylation at Serine-1981 (ATM-pS1981) [1] . Once activated, ATM-pS1981 phosphorylates various downstream substrates such as histone H2AX (H2AX), nibrin (Nbs1), BRCA1, cell-cycle checkpoint kinases Chk1 and Chk2, and p53 that exert vital DNA-damage functions including regulation of cell-cycle checkpoints or inducing repair of damaged DNA or promoting apoptosis through p53 (refs 2 , 3 ). The p53 tumour suppressor protein has a central role in the decision of a cell to undergo either cell-cycle arrest or apoptosis after diverse stresses, including DNA damage, hypoxia and the activation of oncogenes [4] , [5] , [6] . The amount and transcriptional activity of p53 is regulated by post-translational modification, such as phosphorylation, sumoylation, neddation and acetylation [7] . Under normal conditions, p53 protein levels are low owing to Hdm2 (human Mdm2)-mediated ubiquitylation and degradation through the proteasome pathway. On DNA damage, DSBs-activated ATM phosphorylates p53 at Serine-15 (p53-pS15) [8] that may inhibit the interaction of p53 with Hdm2 (ref. 9 ), resulting in p53 stabilization. In addition, ATM can activate Chk2 and homeodomain-interacting protein kinase 2 (HIPK2) to phosphorylate p53 at Serine-20 (p53-pS20) [10] and Serine-46 (p53-pS46) [11] , [12] , respectively, in its transactivation domain, which in turn leads to upregulation of the expression of pro-apoptotic genes such as Bax (Bcl2-associated X protein) and Puma (p53-upregulated modulator of apoptosis) [13] . HIPK2 has a critical role in regulating the apoptotic programme induced by DNA damage [11] , [12] , [14] . Notably, it has been shown that mutations in Serine-15 and Serine-20 of human p53 impair its apoptotic activity [15] , and Serine-46 phosphorylation is crucial for p53-mediated apoptosis after DNA damage [16] . Thus, the regulation of ATM-p53 activation is certainly important in DNA damage-triggered apoptosis. However, the upstream signalling mechanisms that regulate p53 stabilization and activity by ATM-mediated phosphorylation are largely unclear. Interestingly, molecular interactions between p53 and FOXO3 (or FOXO3a) have been discovered [17] , [18] , [19] , [20] . FOXO3 is a pivotal transcription factor that regulates the transcription of a number of genes important for modulating cell-cycle control [21] , DNA damage response [22] , [23] , oxidative and nutritional stress [17] , [24] , aging and longevity [25] , [26] , [27] , cellular apoptosis [28] , [29] , [30] and suppression of cancer [31] , [32] , [33] in animal and human cells. Gene knockout findings support FOXOs' essential functions in tumour suppression [34] and the maintenance of the hematopoietic stem cell pool [35] . Although multiple mechanisms have been shown to regulate FOXO3 activity, phosphorylation inhibits FOXO3 nuclear translocation that is essential for its regulation and function. This nuclear exclusion and translocation of FOXO3 into the cytoplasm inhibits FOXO3-dependent transcription. Loss of function of FOXO3 through phosphorylation has been linked to tumourigenesis and poor patient survival in breast cancer [31] , [32] , suggesting that FOXO3 is a key tumour suppressor. Notably, FOXO3 and p53 share a number of similarities in their functions and regulations. Not only do they interact with each other but also they regulate each other's activity or stability. For instance, it has been reported that activation of p53 can suppress FOXO3 transcriptional activity through serum/glucocorticoid-inducible kinase 1 (SGK1) [36] or induce FOXO3 degradation through Mdm2 (ref. 37 ). Under oxidative stress, p53 can inhibit FOXO3 transcriptional activity [20] . Conversely, it has been shown that activated FOXO3 can stabilize p53 and promote p53-dependent apoptosis [18] . However, during DNA damage-induced apoptosis, the regulation of functional interaction between FOXO3 and p53 to coordinate with crucial DNA damage response proteins such as ATM and Chk2 remains largely unknown. Although several important proteins responsible for activation of the p53-mediated apoptosis have been identified, the mechanism by which ATM activates p53 apoptotic signalling has remained elusive. Our recent findings suggest that FOXO3 is essential for activation of the ATM-BRCA1-Rad17 complex that signals the ATM-mediated repair mechanism at early stages of DNA damage [23] . In addition, it has been found that FOXO3 is necessary for the regulation of normal ATM expression to maintain homoeostasis of hematopoietic stem cells [38] . The fact that prolonged activation of FOXO3 by anticancer agents can trigger apoptosis [29] , [30] suggests that FOXO3 may be involved in regulating the ATM-mediated p53 apoptotic signalling pathway at late stages of DNA damage. Because camptothecin (CPT), a topoisomerase-1 inhibitor, can induce DNA damage and activate the ATM-Chk2 apoptotic pathway in cancer cells [39] , [40] , we set out to determine whether FOXO3 has a key role in linking ATM and Chk2 to the p53-mediated apoptosis after CPT-induced DNA damage, and if so, how the ATM-p53 apoptotic machinery is regulated. Here we show that FOXO3 is functionally associated with the ATM–Chk2–p53 complex, and regulates phosphorylation and the formation of ATM–Chk2–p53 complexes at sites of DNA damage that induce apoptosis. Collectively, we suggest a novel network between FOXO3 and the ATM–Chk2–p53-mediated apoptotic programme after DNA damage. FOXO3 interacts with the ATM–Chk2–p53 complex Because p53-pS15 is phosphorylated directly by ATM-pS1981 and our and other recent studies suggest that FOXO3 may be necessary for the regulation of ATM activation on DNA damage [23] , [38] , we investigated whether FOXO3 has an essential role in the regulation of the ATM-mediated Chk2-p53 apoptotic signalling pathway after DNA damage induced by CPT. To assess the effect of CPT on endogenous FOXO3 expression and the levels of p53-pS15/pS20/pS46, ATM-pS1981, Chk2-pT68 and phosphorylated H2AX (γ-H2AX), we treated MCF-7 cells with CPT or control (dimethylsulphoxide (DMSO)) and analysed the levels of these proteins in cell lysates by immunoblotting (IB). We found that the levels of FOXO3, p53-pS15/pS20/pS46, ATM-pS1981, Chk2-pT68 and γ-H2AX were increased significantly 1–4 h post treatment with CPT, whereas total expressions of Chk2, ATM and H2AX remained unchanged and the control vehicle did not alter the levels of the tested proteins ( Supplementary Fig. S1 ). In addition, other DNA-damaging agents such as etoposide (VP16), ionizing radiation and ultraviolet showed similar results to those of CPT ( Supplementary Fig. S1 ). To validate the interaction between FOXO3 and Chk2 or p53 after DNA damage, we compared the levels of FOXO3, Chk2 and p53 using co-immunoprecipitation (co-IP) and IB assays with cell lysates obtained from MCF-7 cells treated for 2–4 h with CPT. We found that FOXO3 was associated with not only Chk2 and p53 but also p53-pS15 specifically, a direct phosphorylation target of activated ATM, suggesting that FOXO3 may interact with ATM-pS1981 also. Indeed, we showed that FOXO3 was physically associated with p53-pS15, p53-pS20, p53-pS46 (p53-pS15/pS20/pS46), ATM-pS1981, Chk2, HIPK2 and γ-H2AX in cells treated with CPT ( Fig. 1 ). In addition, the expression of HIPK2 was induced after CPT treatment. Collectively, these results suggest that FOXO3 may have a role in regulating the ATM–Chk2–p53 pathway after critical DNA damage. 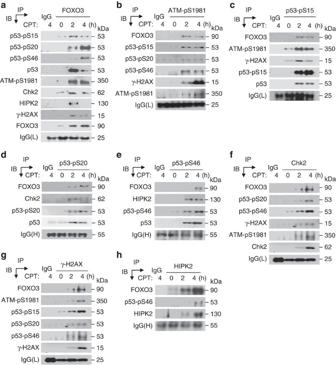Figure 1: FOXO3 interacts with the ATM–Chk2–p53–H2AX complex. (a) Whole-cell lysates of MCF-7 treated with CPT (1 μM) for 2 or 4 h or DMSO (0, control) were subjected to immunoprecipitation (IP) with an anti-FOXO3 antibody (Ab) or an isotype IgG (control) followed by immunoblotting (IB) with Abs as indicated, or an anti-FOXO3 (IP control) or a control Ab against IgG light chain (L). (b–h) Similarly, cell lysates were subjected to IP with an Ab against ATM-pS1981 (b), p53-pS15 (c),p53-pS20 (d), p53-pS46 (e),Chk2 (f), γ-H2AX (g), HIPK2 (h) or an isotype IgG followed by IB with the indicated Abs or a control Ab against IgG(L) or heavy chain (H). Figure 1: FOXO3 interacts with the ATM–Chk2–p53–H2AX complex. ( a ) Whole-cell lysates of MCF-7 treated with CPT (1 μM) for 2 or 4 h or DMSO (0, control) were subjected to immunoprecipitation (IP) with an anti-FOXO3 antibody (Ab) or an isotype IgG (control) followed by immunoblotting (IB) with Abs as indicated, or an anti-FOXO3 (IP control) or a control Ab against IgG light chain (L). ( b – h ) Similarly, cell lysates were subjected to IP with an Ab against ATM-pS1981 ( b ), p53-pS15 ( c ),p53-pS20 ( d ), p53-pS46 ( e ),Chk2 ( f ), γ-H2AX ( g ), HIPK2 ( h ) or an isotype IgG followed by IB with the indicated Abs or a control Ab against IgG(L) or heavy chain (H). Full size image To confirm the sub-cellular locations of FOXO3, p53-pS15/pS20/pS46, ATM-pS1981, Chk2-pT68 and γ-H2AX in the CPT-treated cells, we performed IB analysis with cytoplamic and nuclear extracts from cells treated with CPT and showed that the levels of FOXO3, p53-pS15/pS20/pS46, ATM-pS1981 and γ-H2AX were elevated in the nucleus ( Supplementary Fig. S2 ). These results suggest that DNA damaging agents such as CPT can substantially induce FOXO3 expression and promote ATM and p53 activation in the nucleus concurrently. FOXO3 is co-localized with ATM–Chk2–p53–H2AX nuclear foci An important question in this study is the cellular location of DNA damage-induced FOXO3. In light of the significance of DNA damage-induced FOXO3 interaction with p53-pS15/pS20/pS46, γ-H2AX, ATM-pS1981 and Chk2-pT68, it was plausible to examine whether FOXO3 was recruited to the damaged DNA sites after DNA damage. Thus, we induced spatially localized DSBs in MCF-7 cells by using focused laser micro-irradiation as described previously [41] , [42] . This technique allowed us to detect the recruitment of a unique fraction of FOXO3 and γ-H2AX and/or ATM-pS1981 to the laser-induced DNA damage tracks ( Fig. 2a ). In addition, to determine the physical associations between FOXO3 and p53-pS15/pS20/pS46 or γ-H2AX or ATM-pS1981 or Chk2-pT68 at the sites of DNA lesions, we assessed whether FOXO3 localized to the potential sites of DSBs by co-localization with p53-pS15/pS20/pS46, γ-H2AX, ATM-pS1981 or Chk2-pT68 following CPT-induced DNA damage. MCF-7 cells were treated with CPT or control and stained with specific antibodies. We found that approximately 70–80% of FOXO3 located in the nucleus and co-localized with p53-pS15/pS20/pS46, ATM-pS1981, γ-H2AX and Chk2-pT68 to form nuclear foci after exposure to a low dose of CPT for 2 h, whereas FOXO3 primarily resided in the cytoplasm of cells treated with control ( Fig. 2b–f ; Supplementary Fig. S3 ). To generalize these results, we performed the same experiments in another p53 wild-type (WT) cell line A549 and showed that FOXO3 co-localized with p53-pS15/pS20/pS46, ATM-pS1981, γ-H2AX and Chk2-pT68 to form nuclear foci in A549 cells after CPT treatment ( Supplementary Figs S3 and S4 ), suggesting that FOXO3 may co-localize with p53-pS15/pS20/pS46, ATM-pS1981, γ-H2AX and Chk2-pT68 to sites of DNA breaks in response to DNA damage. 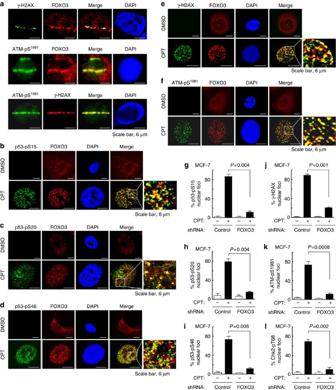Figure 2: FOXO3 is essential for the formation of ATM–Chk2–p53–H2AX nuclear foci. (a) Accumulation of a fraction of FOXO3 at laser-induced damage was detected in MCF-7 cells 30 min after focused laser micro-irradiation. The cells were stained with antibodies (Abs) against FOXO3 and γ-H2AX or ATM-pS1981, followed by fluorescence microscopy as described in the section of Immunofluorescence under 'Methods'. DAPI was used to show the nuclei, and co-localizations of FOXO3 with ATM-pS1981 were shown as the merged images. Scale bar, 6 μm. (b–f) MCF-7 cells were treated with CPT (1 μM) or DMSO control for 2 h, and co-localizations between FOXO3 and p53-pS15 (b), p53-pS20 (c), p53-pS46 (d), γ-H2AX (e) or ATM-pS1981 (f) were detected using Abs as indicated and followed by fluorescence microscopy. Scale bar, 6 μm. (g–l) FOXO3 is necessary for the formation of p53-pS15, p53-pS20 and p53-pS46, γ-H2AX, ATM-pS1981 and Chk2-pT68 nuclear foci on CPT-induced DNA damage. MCF-7 stable cell lines transfected with FOXO3-shRNA or control-shRNA were treated with CPT (1 μM) or DMSO for 2 h, and then the sub-cellular localizations and co-localization of FOXO3 and p53-pS15 (g), p53-pS20 (h), p53-pS46 (i), γ-H2AX (j), ATM-pS1981 (k) or Chk2-pT68 (l) were detected using specific Abs as indicated. An average of 200 cells with specific nuclear foci in each comparison was determined and shown. The images of nuclear foci of these proteins were shown inSupplementary Fig. S5. The error bars represent standard deviation, and the statistical test is the pairedt-test. Figure 2: FOXO3 is essential for the formation of ATM–Chk2–p53–H2AX nuclear foci. ( a ) Accumulation of a fraction of FOXO3 at laser-induced damage was detected in MCF-7 cells 30 min after focused laser micro-irradiation. The cells were stained with antibodies (Abs) against FOXO3 and γ-H2AX or ATM-pS1981, followed by fluorescence microscopy as described in the section of Immunofluorescence under 'Methods'. DAPI was used to show the nuclei, and co-localizations of FOXO3 with ATM-pS1981 were shown as the merged images. Scale bar, 6 μm. ( b – f ) MCF-7 cells were treated with CPT (1 μM) or DMSO control for 2 h, and co-localizations between FOXO3 and p53-pS15 ( b ), p53-pS20 ( c ), p53-pS46 ( d ), γ-H2AX ( e ) or ATM-pS1981 ( f ) were detected using Abs as indicated and followed by fluorescence microscopy. Scale bar, 6 μm. ( g – l ) FOXO3 is necessary for the formation of p53-pS15, p53-pS20 and p53-pS46, γ-H2AX, ATM-pS1981 and Chk2-pT68 nuclear foci on CPT-induced DNA damage. MCF-7 stable cell lines transfected with FOXO3-shRNA or control-shRNA were treated with CPT (1 μM) or DMSO for 2 h, and then the sub-cellular localizations and co-localization of FOXO3 and p53-pS15 ( g ), p53-pS20 ( h ), p53-pS46 ( i ), γ-H2AX ( j ), ATM-pS1981 ( k ) or Chk2-pT68 ( l ) were detected using specific Abs as indicated. An average of 200 cells with specific nuclear foci in each comparison was determined and shown. The images of nuclear foci of these proteins were shown in Supplementary Fig. S5 . The error bars represent standard deviation, and the statistical test is the paired t -test. Full size image FOXO3 is essential for forming ATM–Chk2–p53 nuclear foci Although nuclear foci of p53-pS15, p53-pS20, p53-pS46, γ-H2AX, ATM-pS1981 and Chk2-pT68 were formed significantly (around 65–75%) in the presence of FOXO3 in MCF-7 stable cell line transfected with control-short hairpin RNA (shRNA) after exposure to a low dose (1 μM) of CPT for 2 h, the formations of p53-pS15, p53-pS20, p53-pS46, γ-H2AX, ATM-pS1981 and Chk2-pT68 nuclear foci were greatly reduced in MCF-7 stable cell line transfected with FOXO3-shRNA following the same CPT treatment ( Fig. 2g–l ; Supplementary Fig. S5 ). To show the generality of this effect, we performed the same experiments in A549 cells by treating A549 (control-shRNA) and A549 (FOXO3-shRNA) cells with CPT and showed that knockdown of FOXO3 expression in A549 cells abrogated the formations of p53-pS15, p53-pS20, p53-pS46, γ-H2AX, ATM-pS1981 and Chk2-pT68 nuclear foci in A549 cells following CPT treatment ( Supplementary Figs S6 and S7 ). These results suggest that FOXO3 may be crucial for the formation of p53-pS15, p53-pS20, p53-pS46, γ-H2AX, ATM-pS1981 and Chk2-pT68 nuclear foci after DNA damage induced by CPT. ATM–Chk2–p53–H2AX phosphorylation requires FOXO3 Next, we determined whether silencing of FOXO3 alters the expression or phosphorylation of ATM, Chk2, p53 and H2AX following DNA damage by biochemical approaches. We treated MCF-7 (control-shRNA) and MCF-7 (FOXO3-shRNA) cells with a low dose of CPT for 4 h and performed IB analysis. Interestingly, silencing of FOXO3 did not change the expression of ATM, Chk2, H2AX and p53 total proteins but, significantly, did reduce the levels of phosphorylation (or activation) of ATM, Chk2, p53 and H2AX ( Fig. 3a ). To demonstrate the generality of this finding, we performed the same experiments in A549 cells by treating A549 (control-shRNA) and A549 (FOXO3-shRNA) cells with CPT and performing IB analysis. In agreement with our results in MCF-7 cells, silencing of FOXO3 expression in A549 cells significantly reduced phosphorylation of ATM, Chk2, p53 and H2AX in A549 cells after CPT treatment ( Fig. 3b ), suggesting that indeed FOXO3 is required for ATM–Chk2–p53–H2AX activation in A549 cells on DNA damage. In addition, we have carried out similar experiments in a p53-deficient cell line H1299 by treating H1299 (control-shRNA) and H1299 (FOXO3-shRNA) cells with CPT as described above. We showed that knockdown of FOXO3 expression in H1299 cells diminished phosphorylation of ATM, Chk2 and H2AX in H1299 cells after CPT treatment ( Fig. 3c ), suggesting that FOXO3 is necessary for ATM-Chk2-H2AX activation in H1299 cells following DNA damage. Collectively, these results suggest that FOXO3 is essential for phosphorylation or activation of ATM, Chk2, p53 and H2AX when DNA damage occurs. 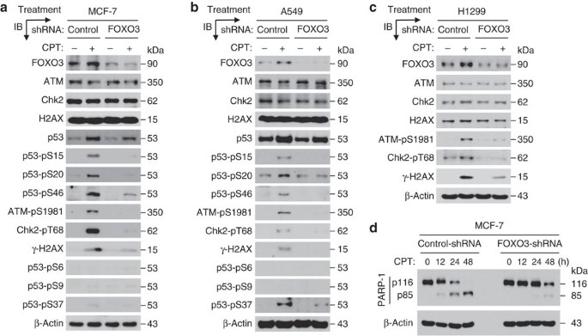Figure 3: FOXO3 is required for ATM–Chk2–p53 phosphorylation and PARP-1 cleavage. (a) MCF-7 stable cell lines transfected with FOXO3-shRNA or control-shRNA were treated with CPT (1 μM) or DMSO (negative control) for 4 h, and whole-cell lysates were prepared and the levels of proteins were analysed by IB with specific antibodies (Abs) as highlighted or an anti-β-actin (loading control). (b,c) A549 (b) and H1299 (c) stable cell lines transfected with FOXO3-shRNA or control-shRNA were treated with CPT (1 μM) or DMSO (negative control) for 4 h, and whole-cell lysates were analysed by IB with specific Abs as indicated or an anti-β-actin. (d) Cell lysates from MCF-7 stable cell lines (FOXO3-shRNA and control-shRNA) treated with CPT (1 μM) for an indicated time course were subjected to IB analysis using Abs against PARP-1 and β-actin (loading control). Figure 3: FOXO3 is required for ATM–Chk2–p53 phosphorylation and PARP-1 cleavage. ( a ) MCF-7 stable cell lines transfected with FOXO3-shRNA or control-shRNA were treated with CPT (1 μM) or DMSO (negative control) for 4 h, and whole-cell lysates were prepared and the levels of proteins were analysed by IB with specific antibodies (Abs) as highlighted or an anti-β-actin (loading control). ( b , c ) A549 ( b ) and H1299 ( c ) stable cell lines transfected with FOXO3-shRNA or control-shRNA were treated with CPT (1 μM) or DMSO (negative control) for 4 h, and whole-cell lysates were analysed by IB with specific Abs as indicated or an anti-β-actin. ( d ) Cell lysates from MCF-7 stable cell lines (FOXO3-shRNA and control-shRNA) treated with CPT (1 μM) for an indicated time course were subjected to IB analysis using Abs against PARP-1 and β-actin (loading control). Full size image FOXO3 is necessary for inducing DNA damage-induced apoptosis To examine the role of FOXO3 in DNA damage-induced apoptosis, we treated MCF-7 cells with a low dose of CPT and analysed apoptosis by the standard poly-ADP-ribose polymerase (PARP) degradation, an indicator of apoptosis [43] and terminal deoxynucleotidyl transferase dUTP nick end labelling (TUNEL) apoptosis assays. We showed that CPT treatment induced significant PARP-1 degradation and TUNEL-positive cells ~8 h post drug treatment, respectively ( Fig. 3d ). Furthermore, we showed that silencing of FOXO3 expression in these cells significantly attenuated this CPT-induced apoptosis ( Figs 3d and 4a,b ), suggesting that FOXO3 may be necessary for promoting apoptosis after DNA damage. To determine whether FOXO3 knockdown also contributes to survival, we treated MCF-7 (control-shRNA) and MCF-7 (FOXO3-shRNA) cells with various doses of CPT or DMSO (control) for 24 h or with 0.25 μM CPT for a time course, and performed cell survival assays by cell counting or the 3-(4,5-dimethylthiazol-2-yl)-2,5-diphenyltetrazolium bromide (MTT) assays. We found that FOXO3 knockdown in these cells significantly promoted survival after CPT treatment ( Fig. 4c,d ). To generalize these results, we compared the survival rates in A549 (control-shRNA) versus A549 (FOXO3-shRNA) cells and H1299 (control-shRNA) versus H1299 (FOXO3-shRNA) cells following CPT treatment. We showed that silencing of FOXO3 in these cells significantly enhanced survival after CPT treatment ( Supplementary Fig. S8 ). Taken together, these results suggest that FOXO3 is essential for regulating survival and apoptosis when DNA damage occurred. 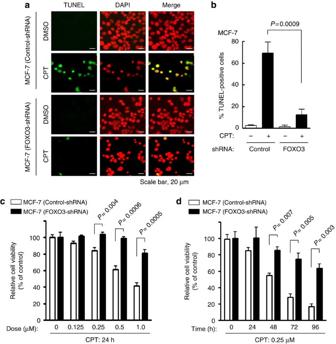Figure 4: FOXO3 is necessary for inducing DNA damage-induced apoptosis. (a) MCF-7 stable cell lines (FOXO3-shRNA and control-shRNA) were treated with CPT (1 μM) or DMSO (control) for 48 h, and the cells were fixed on the slides for determining cellular apoptosis by TUNEL assays (Promega). Nuclei were stained with DAPI (colour-inverted to red), and merged images (yellow) were considered as apoptotic cells. Scale bar, 20 μm. (b) An average (%) of apoptotic (TUNEL-positive) cells was determined and shown in the diagram; the samples include three biological replicates, the error bars represent standard deviation, and the statistical test is the pairedt-test. The significantP-values between the FOXO3-shRNA group versus the control group treated with CPT are highlighted. (c,d) MCF-7 (control-shRNA) and MCF-7 (FOXO3-shRNA) cells were treated with various doses of CPT or DMSO (control) for 24 h (c) or with a low dose CPT (0.25 μM) for a time course as indicated (d), and performed cell survival assays by the MTT assays (c) or cell counting (d). The significantP-values between the FOXO3-shRNA group versus the control group treated with CPT are indicated. The number of biological replicates is three, the error bars represent standard deviation, and the statistical test is the pairedt-test. Figure 4: FOXO3 is necessary for inducing DNA damage-induced apoptosis. ( a ) MCF-7 stable cell lines (FOXO3-shRNA and control-shRNA) were treated with CPT (1 μM) or DMSO (control) for 48 h, and the cells were fixed on the slides for determining cellular apoptosis by TUNEL assays (Promega). Nuclei were stained with DAPI (colour-inverted to red), and merged images (yellow) were considered as apoptotic cells. Scale bar, 20 μm. ( b ) An average (%) of apoptotic (TUNEL-positive) cells was determined and shown in the diagram; the samples include three biological replicates, the error bars represent standard deviation, and the statistical test is the paired t -test. The significant P -values between the FOXO3-shRNA group versus the control group treated with CPT are highlighted. ( c , d ) MCF-7 (control-shRNA) and MCF-7 (FOXO3-shRNA) cells were treated with various doses of CPT or DMSO (control) for 24 h ( c ) or with a low dose CPT (0.25 μM) for a time course as indicated ( d ), and performed cell survival assays by the MTT assays ( c ) or cell counting ( d ). The significant P -values between the FOXO3-shRNA group versus the control group treated with CPT are indicated. The number of biological replicates is three, the error bars represent standard deviation, and the statistical test is the paired t -test. Full size image FOXO3 may need ATM–Chk2–p53 activation to lead to apoptosis Further, to determine the roles of phosphorylated ATM–Chk2–p53 in the regulation of FOXO3-mediated apoptosis following DNA damage induced by CPT, we transfected MCF-7 cells with control-short interfering RNA (siRNA) or siRNA-targeting ATM, Chk2 or p53, and treated these cells with a low dose of CPT. Markedly, silencing the expression of ATM, Chk2 or p53 with specific siRNAs in MCF-7 cells abolished CPT-induced PARP-1 degradation ( Fig. 5a ), suggesting that ATM–Chk2–p53 proteins are necessary for the FOXO3-mediated apoptosis on CPT-induced DNA damage. In addition, we treated MCF-7 cells with specific inhibitors of ATM, Chk2 and p53 or control for 6 h before exposure to a low dose of CPT or control, and we showed that inhibiting the activity of ATM, Chk2 or p53 significantly diminished the levels of ATM-pS1981, Chk2-pT68 or p53 phosphorylated isoforms (p53-pS15/pS20/pS46) and abrogated CPT-induced PARP-1 degradation ( Fig. 5b ). As controls, we showed that these inhibitor treatments did not alter FOXO3 expression significantly; thus, the lack of PARP-1 degradation could not be attributed to attenuation of FOXO3 expression in these cells. These results suggest that the activities of ATM-pS1981-, Chk2-pT68- and p53-phosphorylated isoforms (p53-pS15/pS20/pS46) may be essential for FOXO3-mediated apoptosis. 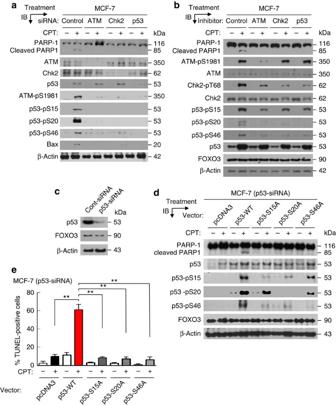Figure 5: Phosphorylated ATM–Chk2–p53 may be needed for FOXO3-mediated apoptosis. (a) MCF-7 cells were transfected with control-siRNA (control) or siRNA (0.3 μM) targeting ATM, Chk2 or p53 and incubated for 48 h, and then these cells were treated with CPT (1 μM) (+) or DMSO (−) for 48 h. Whole-cell lysates were prepared from these treated cells and the levels of PARP-1 and its degraded proteins, ATM, Chk2, p53 and their phosphorylated proteins or a p53 target (Bax) were analysed by IB with specific antibodies (Abs) as indicated or an anti-β-actin (loading control). (b) MCF-7 cells were first treated with ATM inhibitor (Mirin) or Chk2 inhibitor (NSC10955) or p53 inhibitor (Pifithrin), 20 μM of each, or DMSO for 6 h, and then treated with CPT (1 μM) or DMSO for 16 h. Whole-cell lysates were prepared from these treated cells and the levels of PARP-1 and its degraded proteins, and the indicated proteins and β-actin were analysed by IB analysis with specific Abs. (c) MCF-7 cells were transfected with p53-siRNA or Cont-siRNA (Control-siRNA) for 48 h. Whole-cell lysates were prepared from these transfected cells and the expressions of p53 and FOXO3 (control) were determined by IB analysis with specific Abs. (d) MCF-7 (p53-siRNA) cells were transfected with pcDNA3 (control) or p53 wild-type (WT) or mutant (p53-S15A or p53-S20A or p53-46A) expression vectors (2 μg DNA for each) for 48 h, and then treated with CPT (1 μM) (+) or DMSO (−) for 48 h. Whole-cell lysates were prepared from these treated cells and the levels of PARP-1 and its degraded proteins, and the indicated proteins were analysed by IB analysis with specific Abs. (e) MCF-7 (p53-siRNA) cells were transfected with control and expression vectors for 24 h, the transfected cells were treated with CPT (1 μM) or DMSO control for 36 h, and cellular apoptosis was determined by TUNEL assays (Promega). Images of apoptotic cells were shown inSupplementary Fig. S9. An average (%) of TUNEL-positive (apoptotic) cells was determined and shown in the diagram. **P=0.0001 (pairedt-test). Figure 5: Phosphorylated ATM–Chk2–p53 may be needed for FOXO3-mediated apoptosis. ( a ) MCF-7 cells were transfected with control-siRNA (control) or siRNA (0.3 μM) targeting ATM, Chk2 or p53 and incubated for 48 h, and then these cells were treated with CPT (1 μM) (+) or DMSO (−) for 48 h. Whole-cell lysates were prepared from these treated cells and the levels of PARP-1 and its degraded proteins, ATM, Chk2, p53 and their phosphorylated proteins or a p53 target (Bax) were analysed by IB with specific antibodies (Abs) as indicated or an anti-β-actin (loading control). ( b ) MCF-7 cells were first treated with ATM inhibitor (Mirin) or Chk2 inhibitor (NSC10955) or p53 inhibitor (Pifithrin), 20 μM of each, or DMSO for 6 h, and then treated with CPT (1 μM) or DMSO for 16 h. Whole-cell lysates were prepared from these treated cells and the levels of PARP-1 and its degraded proteins, and the indicated proteins and β-actin were analysed by IB analysis with specific Abs. ( c ) MCF-7 cells were transfected with p53-siRNA or Cont-siRNA (Control-siRNA) for 48 h. Whole-cell lysates were prepared from these transfected cells and the expressions of p53 and FOXO3 (control) were determined by IB analysis with specific Abs. ( d ) MCF-7 (p53-siRNA) cells were transfected with pcDNA3 (control) or p53 wild-type (WT) or mutant (p53-S15A or p53-S20A or p53-46A) expression vectors (2 μg DNA for each) for 48 h, and then treated with CPT (1 μM) (+) or DMSO (−) for 48 h. Whole-cell lysates were prepared from these treated cells and the levels of PARP-1 and its degraded proteins, and the indicated proteins were analysed by IB analysis with specific Abs. ( e ) MCF-7 (p53-siRNA) cells were transfected with control and expression vectors for 24 h, the transfected cells were treated with CPT (1 μM) or DMSO control for 36 h, and cellular apoptosis was determined by TUNEL assays (Promega). Images of apoptotic cells were shown in Supplementary Fig. S9 . An average (%) of TUNEL-positive (apoptotic) cells was determined and shown in the diagram. ** P =0.0001 (paired t -test). Full size image Next, we transfected the MCF-7 p53-knockdown, MCF-7 (p53-siRNA) ( Fig. 5c ), cells with pcDNA3 (control) or p53-WT or mutant (p53-S15A or p53-S20A or p53-46A) expression vectors for 48 h, and then treated them with a low dose (1 μM) of CPT or control for 48 h. Interestingly, over-expression of p53-WT-promoted CPT-induced PARP-1 degradation and apoptosis, whereas over-expression of p53-S15A, p53-S20A or p53-S46A mutant failed to induce PARP-1 degradation and TUNEL apoptosis after CPT treatment ( Fig. 5d,e ; Supplementary Fig. S9 ). As controls, we showed that over-expression of these p53 mutants did not significantly change FOXO3 expression, suggesting that the observed negative effect on PARP-1 degradation or TUNEL apoptosis cannot be ascribed to debilitation of FOXO3 in these cells. In addition, we repeated the same experiments in another p53-null cell line, H1299, and obtained the same reproducible results ( Supplementary Fig. S10 ), confirming that these p53 phosphorylated isoforms (p53-pS15/pS20/pS46) are necessary for FOXO3-mediated apoptosis following DNA damage induced by CPT. Collectively, these results suggest that FOXO3 may require ATM–Chk2–p53 phosphorylated isoforms to lead to apoptosis after DNA damage. FOXO3 regulates chromatin retention of phosphorylated p53 An important question in mechanism is how FOXO3 contributes to the activation of ATM-pS1981, Chk2-pT68 and p53-pS15/pS20/pS46 in cells on DNA damage. Hence, we sought to determine whether FOXO3 is required for binding and retention of ATM-pS1981, Chk2-pT68 and p53-pS15/pS20/pS46 proteins to the chromatin following DNA damage. We treated MCF-7 (control-shRNA) and MCF-7 (FOXO3-shRNA) cells with a low dose of CPT for 4 h and performed chromatin retention assays. Remarkably, silencing of FOXO3 expression in MCF-7 cells significantly diminished chromatin retention of ATM-pS1981, Chk2-pT68, p53-pS15/pS20/pS46 and γ-H2AX ( Fig. 6a ), suggesting that FOXO3 may have a role in regulating chromatin retention of phosphorylated ATM–Chk2–p53–H2AX. 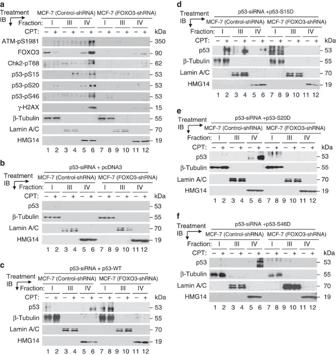Figure 6: FOXO3 has a role in regulating chromatin retention of phosphorylated p53. (a) MCF-7 stable cell lines transfected with FOXO3-shRNA or control-shRNA were treated with CPT (1 μM) (+) or DMSO (−) (control) for 4 h, and cells were collected and fractionated with Nonidet P-40 as described in the section of Chromatin Retention Assay under 'Methods'. Equal amount (20 μg) of each fraction was analysed by IB analysis with the highlighted antibodies as described above. Proteins β-tubulin, lamin A/C and HMG14 (high-mobility-group 14, a chromosome-binding protein) represent the fractionation and loading controls of the cytosol (fraction I), the nucleoplasm (fraction III) and the chromatin (fraction IV), respectively. (b–f) MCF-7 (control-shRNA) and MCF-7 (FOXO3-shRNA) cells were transfected with p53 siRNA for 48 h, then transfected with pcDNA3 (negative control) (b) or the p53-WT vector (c) or the specific vectors expressing p53-S15D (d), p53-S20D (e) and p53-S46D (f) for 36 h. The transfected cells were treated with CPT (1 μM) or DMSO for 4 h, then cells were collected and subjected to chromatin fractionation and IB analysis as described above. Figure 6: FOXO3 has a role in regulating chromatin retention of phosphorylated p53. ( a ) MCF-7 stable cell lines transfected with FOXO3-shRNA or control-shRNA were treated with CPT (1 μM) (+) or DMSO (−) (control) for 4 h, and cells were collected and fractionated with Nonidet P-40 as described in the section of Chromatin Retention Assay under 'Methods'. Equal amount (20 μg) of each fraction was analysed by IB analysis with the highlighted antibodies as described above. Proteins β-tubulin, lamin A/C and HMG14 (high-mobility-group 14, a chromosome-binding protein) represent the fractionation and loading controls of the cytosol (fraction I), the nucleoplasm (fraction III) and the chromatin (fraction IV), respectively. ( b – f ) MCF-7 (control-shRNA) and MCF-7 (FOXO3-shRNA) cells were transfected with p53 siRNA for 48 h, then transfected with pcDNA3 (negative control) ( b ) or the p53-WT vector ( c ) or the specific vectors expressing p53-S15D ( d ), p53-S20D ( e ) and p53-S46D ( f ) for 36 h. The transfected cells were treated with CPT (1 μM) or DMSO for 4 h, then cells were collected and subjected to chromatin fractionation and IB analysis as described above. Full size image To demonstrate the important role of FOXO3 in regulating chromatin retention of the activated p53 proteins in a phosphorylation-independent manner, we silenced endogenous p53 in MCF-7 (control-shRNA) and MCF-7 (FOXO3-shRNA) cells with p53 siRNA as described above. We then transfected these p53-knockdown cells with pcDNA3 (negative control) or the p53-WT vector or the specific vectors expressing p53-S15D, p53-S20D and p53-S46D, which are the constitutively activated mutant p53 proteins with the specific Serine (S) residue being mutated to Aspartic acid (D) that mimics the phosphorylated-S residue [16] , [44] , [45] , for 36 h. We treated these transfected cells with a low dose of CPT for 4 h, then harvested cells and performed chromatin fractionation as described above. Remarkably, silencing FOXO3 significantly diminished chromatin retention of these p53-S15D, p53-S20D and p53-S46D proteins ( Fig. 6d–f ), suggesting that FOXO3 may have a necessary role in chromatin retention of the activated p53 proteins independent of their phosphorylation. ATM is a key DNA damage sensor that has a central role in controlling the DNA damage response. A great deal of information has been obtained on the DNA-damage sensor mechanisms detecting DSBs in recent years; however, it is still unclear how specific DNA lesions are recognized and how signalling is delivered downstream to the apoptotic machinery [1] , [2] , [3] . It also remains largely unknown when the sensor proteins should signal repair mechanisms to repair damaged DNA and when they would trigger apoptosis. Although activation of the p53-mediated apoptosis has a critical role in tumour suppression, the control of activation of ATM–Chk2–p53 apoptotic signalling is unclear [4] , [5] , [6] , [7] , [8] , [9] , [10] , [11] , [12] . In this study, we show a critical role of FOXO3 in regulating the formation of ATM-pS1981-Chk2-p53-pS15/pS20/pS46 complexes at sites of DNA breaks, and its role in promoting the ATM–Chk2–p53 apoptotic-signalling pathway after DNA damage. Our findings suggest that FOXO3 may be important for regulating chromatin retention of these phosphorylated (and/or activated) ATM–Chk2–p53 proteins in the nucleus when DNA damage occurs. Although it is possible that the general abundance of the proteins examined may regulate the levels of protein–protein interaction and chromatin retention observed here, our data show specific interactions between FOXO3 and p53-pS15 or p53 and the extent of these interactions in co-IP is significantly lower at 4 h than at 2 h after CPT treatment ( Fig. 1a,c ), whereas the levels of FOXO3 and p53-pS15 are considerably higher at 4 h than at 2 h post CPT treatment ( Supplementary Fig. S1a ). Taken together, these results clearly indicate that the formation of specific FOXO3/p53-pS15, FOXO3/p53, FOXO3-Chk2 and other complexes (as shown by co-IP) is not solely dependent on the abundance of these proteins examined. Interestingly, it has been shown that p53 activation can downregulate FOXO3 through induction of SGK1 or Hdm2 (refs 36 , 37 ), which in turn promotes ubiquitin-dependent degradation of p53 (ref. 46 ). These intriguing findings suggest the possible roles of p53 and Hdm2 (refs 37 , 47 ) in downregulation of FOXO3 as negative feedback loops. On the other hand, it has been reported that activation of ATM can enhance p53 stabilization by direct phosphorylation of Hdm2 (refs 48 , 49 ) and inhibition of its RING domain oligomerization and E3 ligase [50] . Collectively, we have proposed a schematic representation of the FOXO3-dependent phosphorylation or activation of ATM-pS1981/p53-pS15, Chk2-pT68/p53-pS20 and HIPK2/p53-pS46 together with their negative feedback loops and the downstream p53 apoptotic-signalling pathways after DNA damage ( Fig. 7 ). 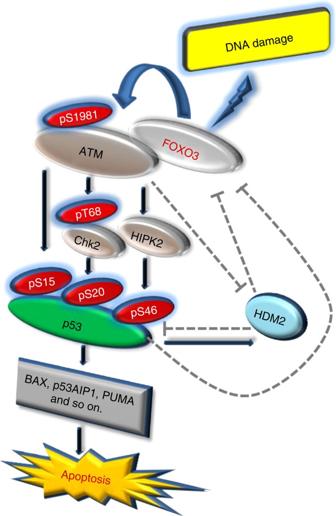Figure 7: A link between FOXO3 and the ATM–Chk2–p53-mediated apoptotic programme. A schematic shows the FOXO3-dependent activation of ATM-pS1981, Chk2-pT68, HIPK2, p53-pS15, p53-pS20, p53-pS46 and the possible roles of p53 and Hdm2 in downregulation of FOXO3 as negative feedback loops, and the downstream p53 apoptotic-signalling pathway after DNA damage induced by CPT. The dashed lines denote the inhibitory pathways according to the published literature. Figure 7: A link between FOXO3 and the ATM–Chk2–p53-mediated apoptotic programme. A schematic shows the FOXO3-dependent activation of ATM-pS1981, Chk2-pT68, HIPK2, p53-pS15, p53-pS20, p53-pS46 and the possible roles of p53 and Hdm2 in downregulation of FOXO3 as negative feedback loops, and the downstream p53 apoptotic-signalling pathway after DNA damage induced by CPT. The dashed lines denote the inhibitory pathways according to the published literature. Full size image At the early stages of DNA damage with low levels of DSBs, it is possible that only a minor fraction of p53 is activated that is sufficient to drive the transcription of the p21Cip1 gene, resulting in cell-cycle arrest. However, with high levels of DSBs, p53 is activated and accumulated above a particular threshold that upregulates the expression of pro-apoptotic genes such as Bax, Puma and p53AIP1 (p53-regulated apoptosis-inducing protein 1) [13] , [51] . Although CPT can significantly upregulate the expression of these p53 downstream target genes in the presence of FOXO3, we have found that the expression levels of Bax, Puma and p53AIP1 were significantly reduced in the FOXO3-knockdown MCF-7 cells after CPT treatment (data not shown), suggesting that CPT induces these pro-apoptotic proteins in a FOXO3-dependent manner. It has been shown that phosphorylation of p53-pS46 is activated by HIPK2 kinase. Although HIPK2 has been found to be a downstream target of ATM [12] , it is unclear how DNA damage induces the ATM-HIPK2-p53-pS46 signalling pathway. In this study, we show that CPT-induced DNA damage can induce the FOXO3-dependent phosphorylation of ATM-pS1981 and p53-pS46 and the interactions of FOXO3-HIPK2-p53-pS46, suggesting that FOXO3 may have a critical role in activation of the ATM-HIPK2-p53-pS46 signalling pathway and provide an essential link between ATM-pS1981 and p53-pS15/pS20/pS46 simultaneously on DNA damage. In addition, we show that FOXO3 is necessary for inducing DNA damage-induced apoptosis. Taken together, these results suggest that FOXO3 has an essential role in the regulation of ATM-p53-mediated apoptosis after DNA damage. Moreover, we have found that ATM-pS1981, Chk2-pT68 and p53 phosphorylated isoforms (p53-pS15/pS20/pS46) are essential for FOXO3-mediated apoptosis following DNA damage. To the best of our knowledge, this is the first evidence that FOXO3 requires phosphorylation (or activation) of p53 and its upstream kinases ATM and Chk2 together to lead to apoptosis after DNA damage. Our results are consistent with a recent finding that p53 is necessary for FOXO3 transcriptional upregulation and transactivation in vivo [33] . Because there is no increase in FOXO3 levels in MCF-7 cells after CPT treatment for 16 h ( Fig. 5b ) and 48 h ( Fig. 5d ), we performed IB analysis of FOXO3 and ATM–Chk2–p53 proteins with full time-course of CPT treatment (0–48 h) in MCF-7 cells, and showed that the amount of FOXO3 protein remains at a similar level between 0 and 16 h and between 0 and 48 h after CPT treatment ( Supplementary Fig. S11a ), indicating that these results do not contradict the FOXO3 increase shown in Supplementary Fig. S1a and Fig. 1a . Together, our results suggest that FOXO3 cooperates with the ATM–Chk2–p53 apoptotic programme concurrently, leading to a high degree of activation of the p53-mediated apoptotic pathways following DNA damage. Although it is known that FOXO3 is physically associated with p53 (refs 17 , 18 , 19 , 20 ), the molecular mechanisms underlying FOXO3-mediated regulation of the p53-induced apoptotic pathway on DNA damage and vice versa are largely unknown. Our findings suggest that FOXO3 is required for phosphorylation of p53 isoforms (p53-pS15/pS20/pS46). To further elucidate the mechanism by which FOXO3 regulates p53 activation in the DNA damage response, using the chromatin retention assays, we show that silencing of FOXO3 expression in MCF-7 cells significantly diminishes chromatin retention of p53-pS15/pS20/pS46 on DNA damage ( Fig. 6 ). Moreover, FOXO3 is triggered to migrate markedly to the chromatin from the cytoplasm in parallel with phosphorylated ATM–Chk2–p53 following DNA damage ( Fig. 6a ), suggesting that FOXO3 may cooperate with phosphorylated ATM–Chk2–p53 and migrate to the DSB sites on the chromatin concurrently after DNA damage. To determine whether FOXO3 is still localized to the chromatin at late time treatment with CPT, we performed the same experiments of Fig. 6a at 24 h after CPT treatment and showed that the localization of FOXO3 to the chromatin is significantly reduced after 24 h CPT treatment compared with 4 h ( Supplementary Fig. S11b ). Collectively, these results suggest that FOXO3 contributes to the DNA damage response by controlling phosphorylation of ATM–Chk2–p53 or regulating chromatin retention of these phosphorylated proteins in the nucleus or both. In addition to FOXO3, Mre11-Rad50-Nbs1 (MRN) and other factors can interact with ATM and regulate its kinase activity that enhances its ability to phosphorylate substrates in vitro [52] , [53] . However, the fact that ATM can be activated by ionizing radiation treatment in cells lacking Nbs1 or BRCA1 but cannot be recruited to the DSB sites suggests that the MRN complex may increase the accumulation of ATM at the DSB sites on the chromatin [54] , [55] but other factors can activate ATM activity in an MRN-independent manner. Thus, it is plausible that ATM activity may be regulated by two distinct events, one being the activation of intermolecular autophosphorylation of ATM [56] by multiple factors such as FOXO3 and the MRN complex, and the other, recruitment of the activated ATM to the substrate sites. In this respect, the MRN complex induces the ATM DNA-damage response to facilitate the repair of damaged DNA at early stages of DNA damage [57] , whereas if the damaged DNA cannot be repaired, FOXO3 triggers a cell death programme by promoting the ATM–Chk2–p53 apoptotic mechanism. This orchestrated genome maintenance programme in response to DNA damage stress mediates not only timely DNA repair to avert the most harmful lesions to the integrity of the genome but also an apoptotic mechanism to eliminate cells with heavily damaged genomes, thereby the development of cancerous cells can be prevented [58] . Cell culture and transfection All cell lines were grown at 37 °C and 5% CO 2 in DMEM/F12 supplemented with L -glutamine, penicillin/streptomycin and 10% fetal bovine serum. All siRNAs against ATM (sc-29761), CHK2 (sc-29271), p53 (sc-29435) and control siRNA (sc-44231) were obtained from Santa Cruz Biotechnology (Santa Cruz, CA). Four HuSH 29mer shRNA constructs against human FOXO3 (NM_001455) and control HuSH shRNA cloning vector (pRS) using U6 promoter were purchased from OriGene Technologies, Inc. (Rockville, MD). The oligonucleotide sequences in the shRNA expression cassettes are shown in Supplementary Table S1 . MCF-7 cells were transfected with a combination of four HuSH 29mer shRNA constructs concurrently or control pRS vector by liposome using GenJet In Vitro DNA Tranfection Reagent for MCF-7 Cell (SignaGen Laboratories, Gaithersburg, MD). After puromycin selection (1 μg ml −1 ), the MCF-7 FOXO3-knockdown pooled stable clones (designated MCF-7 (FOXO3-shRNA)) and the vector control stable clones (designated MCF-7 (Control-shRNA)) were selected. Similarly, the A549 or H1299 FOXO3-knockdown pooled stable clones (designated A549 (FOXO3-shRNA) or H1299 (FOXO3-shRNA)) and the vector control stable clones (designated A549 (Control-shRNA) or H1299 (Control-shRNA)) were generated and selected as described above. For transfection with siRNA, MCF-7 cells were transfected with specific siRNA or control siRNA as indicated by using DharmaFECT 1 transfection reagent (Thermo Scientific, Rockford, IL) according to the manufacturer's instructions. Whole-cell lysates were prepared 48 h after transfection as described previously [31] . Antibodies and reagents The DNA damaging agent CPT was purchased from Sigma (St Louis, MO). The drug was dissolved in DMSO and stored in aliquots at −20 °C. Antibodies specific to FOXO3 (FKHRL1, H-144 (1:1,000 dilution) and N-16, 1:500 dilution), PARP (1:1,000 dilution), CHK2 (1:1,000 dilution), p53 (DO-1 and FL-393, 1:1,000 dilution), phospho-p53 (p53-pS15, p53-pS20 and p53-pS46, 1:1,000 dilution), Lamin A/C (1:2,000 dilution) and β-tubulin (1:2,000 dilution) were obtained from Santa Cruz Biotechnology. Antibodies against H2AX (1:2,000 dilution), phospho-H2AX Serine-139 (γ-H2AX, 1:1,000 dilution) and phospho-ATM Serine-1981 (ATM-pS1981, 1:1,000 dilution) were purchased from Millipore (Billerica, MA). Antibodies against phospho-ATM Serine-1981 (ATM-pS1981, 1:1,000 dilution), phospho-Chk2 (Chk2-pT68, 1:1,000 dilution), p53 (1:1,000 dilution), phospho-p53 (p53-pS6, p53-pS9, p53-pS15, p53-pS20, p53-pS37, and p53-pS46, 1:1,000 dilution), Bax (1:500 dilution) and Puma (1:500 dilution) were purchased from Cell Signaling Technology (Danvers, MA). Antibodies against ATM (BL116G, 1:500 dilution) were purchased from Bethyl Laboratories (Montgomery, TX). Antibodies against FOXO3 (3280-1, 2071-1, 1:1,000 dilution) and phospho-ATM Serine-1981 (1:1,000 dilution) were obtained from Epitomics (Burlingame, CA), and an antibody against FKHRL1 (06-951) was obtained from Upstate Biotechnology (Lake Placid, NY). Antibodies against p21Cip1 (1:1,000 dilution) and p27Kip1 (1:1,000 dilution) were purchased from Cell Signaling Technology and/or BD PharMingen (San Diego, CA). Antibody against β-actin (1:3,000 dilution) was purchased from Sigma. Antibody against HMG14 (high-mobility-group 14, 1:2,000 dilution) was purchased from Abcam (Cambridge, MA). Alexa 488-, Alexa 594- and Alexa-647-conjugated secondary antibodies (1:200 dilution) were obtained from Molecular Probes (Eugene, OR). ATM inhibitor (Mirin) and Chk2 inhibitor (NSC10955) were purchased from Santa Cruz Biotechnology, and p53 inhibitor (Pifithrin) was obtained from Tocris Bioscience. MTT was obtained from Invitrogen and DMSO was purchased from Sigma. Laser micro-irradiation and imaging Live MCF-7 cell imaging combined with laser micro-irradiation was described previously [41] , [42] . Briefly, fluorescence data were acquired with an Axiovert 200M microscope (Carl Zeiss MicroImaging, Thornwood, NY). A 365-nm pulsed nitrogen laser (Spectra-Physics, Mountain View, CA) was directly coupled to the epifluorescence path of the microscope. DSBs were introduced in the nucleus by micro-irradiation with 365 nm laser. Cells were recovered for 30 min in the incubator, followed by immunofluorescent staining. Images were taken with an AxioCam HRm camera and fluorescence intensities of micro-irradiated areas were determined by using Axiovision Software, version 4.5 (Carl Zeiss). Immunofluorescence MCF-7 and A549 cells were grown on glass coverslips. After treatment with CPT (1 μM) for 2 or 4 h, cells were fixed with 4 % paraformaldehyde for 10 min and permeabilized with Triton X-100 (0.5%). Slide culture chambers were washed with phosphate-buffered saline (PBS) and blocked with PBS-containing 2% BSA, incubated with an antibody specific to FOXO3, ATM-pS1981, γ-H2AX, p53-pS15, p53-pS20, p53-pS46 or Chk2-pT68 (1:50–1:200 dilution), followed by Alexa 594- or 647 (red)-conjugated anti-rabbit, Alexa 594- (1:200 dilution) or 647 (red)-conjugated anti-goat (1:200 dilution), and Alexa 488 (green)-conjugated anti-mouse (1:200 dilution) or rabbit (1:200 dilution) secondary antibodies (Molecular Probes). Cells were counterstained with 4',6-diamidino-2-phenylindole (DAPI; Sigma) to show the nuclei. Specific staining was visualized and images were captured with a Leica SP2 AOBS confocal laser scanning microscope. To analyse quantitative co-localization, we used ~100 cell images randomly captured by confocal microscopy. The volume and percentage of p53-pS20 co-localized with FOXO3 were measured using the Velocity software (ver. 6.1, Improvision, Perkin-Elmer). To measure foci-positive cells, we used ~200 cells randomly captured by confocal microscopy. The percentages of considering foci-positive cells were calculated from cells containing at least five foci. Each error bar presented is the mean of standard deviation. Immunoprecipitation and immunoblotting All IP experiments were performed as described previously [23] . Briefly, cells were washed twice with PBS and lysed with lysis buffer containing protease inhibitors at 4 °C for 20 min. The lysates were centrifuged at 16,000 g for 10 min to remove cell debris. Total protein concentration was determined as described above. Protein samples were first precleared with a nonspecific IgG antibody. Precleared lysates were then incubated with an antibody by rotating at 4 °C overnight followed by the addition of 25 μl of 50% protein A- or protein G-sepharose slurry and rotating for 1 h. Protein A/G beads were collected and washed with lysis buffer four times. Immunoprecipitates were resolved by 6 or 8% or 10 or 12% SDS–polyacrylamide gel eletrophoresis (PAGE) and analysed by IB analysis. For IB analysis, the protein samples were subjected to SDS–PAGE and transferred onto nitrocellulose membranes (Bio-Rad). Membranes were blocked for 1 h in 3% bovine serum albumin (BSA) in Tris-buffered saline containing 0.1% Tween-20 (TBST) and incubated for 1 h with primary antibody diluted in TBST containing 1% BSA. After three washes with TBST, membranes were incubated for 1 h with horseradish peroxidase-conjugated secondary antibodies (1:3,000 or 1:5,000 dilution) in TBST containing 3% BSA. The immunoblots were visualized by an enhanced chemiluminescence kit obtained from Santa Cruz Biotechnology or West-Q ECL Platinum Solution obtained from GenDEPOT. TUNEL assay Cells were grown on glass coverslips. After treatment with CPT (1 μM) for 48 or 60 h, cells were fixed with 4% paraformaldehyde solution and permeabilized with Triton X-100 (0.2%). For TUNEL assay, cellular apoptosis assay was determined by enzymatic labelling of DNA strand breaks with a TUNEL assay kit (the DeadEnd Fluorometric TUNEL System, Promega) according to the manufacturer's instructions. Nuclei were stained with DAPI (colour was inverted to red). Merged images (yellow) were considered as apoptotic cells and counted under a confocal laser scanning microscope (Leica SP2 AOBS). Chromatin retention assay These experiments were performed as described previously [59] with some modifications. Cells (1×10 7 ) were suspended for 5 min on ice in 150 μl of fractionation buffer (50 mM HEPES, pH 7.5, 150 mM NaCl, 1 mM EDTA) containing 0.2% Nonidet P-40 (Nonidet P-40), supplemented with protease inhibitors (5 μg ml −1 each of pepstatin, leupeptin and aprotonin) and phosphatase inhibitors. Following centrifugation at 1,000 g for 5 min, the supernatant was collected (fraction I) and pellets were washed with the same buffer. After the washing step, the washed sample was collected as before (fraction II), and the nuclear pellets were further extracted for 40 min on ice with 150 μl of fractionation buffer containing 0.5% Nonidet P-40. The extracts were clarified by centrifugation at 16,000 g for 15 min (fraction III). The pellets were finally lysed in fractionation buffer II and boiled for 5 min (fraction IV). After determining the concentration of all fractions, samples were separated on 8% or 10% SDS–PAGE gels and blotted onto nitrocellulose membranes (Boi-Rad). Membranes were blocked for 1 h in 3% BSA in TBST and incubated for 1 h with primary antibody (1:500 or 1:1,000) diluted in TBST containing 1% BSA. After three washes with TBST, membranes were incubated for 1 h with secondary antibodies (1:3,000) in TBST containing 3% BSA. The immunoblots were visualized by an enhanced chemiluminescence kit obtained from GenDEPOT. Statistical analysis All data are expressed as means and standard deviations from at least three determinations. The statistical significance of difference in nuclear co-localization of proteins examined in cells (by immunofluorescence) and the percentage of apoptotic nuclei (by TUNEL assay) between two groups was analysed with two-sided unpaired Student's t -tests when the variances were equal with Grahpad PRISM (Ver.4.02) statistical software (San Diego, CA). All statistical tests were two-sided, and P -values less than 0.05 were considered statistically significant. How to cite this article: Chung, Y. M. et al . FOXO3 signalling links ATM to the p53 apoptotic pathway following DNA damage. Nat. Commun. 3:1000 doi: 10.1038/ncomms2008 (2012).